A correlated nickelate synaptic transistor Inspired by biological neural systems, neuromorphic devices may open up new computing paradigms to explore cognition, learning and limits of parallel computation. Here we report the demonstration of a synaptic transistor with SmNiO 3 , a correlated electron system with insulator–metal transition temperature at 130°C in bulk form. Non-volatile resistance and synaptic multilevel analogue states are demonstrated by control over composition in ionic liquid-gated devices on silicon platforms. The extent of the resistance modulation can be dramatically controlled by the film microstructure. By simulating the time difference between postneuron and preneuron spikes as the input parameter of a gate bias voltage pulse, synaptic spike-timing-dependent plasticity learning behaviour is realized. The extreme sensitivity of electrical properties to defects in correlated oxides may make them a particularly suitable class of materials to realize artificial biological circuits that can be operated at and above room temperature and seamlessly integrated into conventional electronic circuits. Artificial neuromorphic electronics that mimic the working principle of neural synapses implement a unique computing paradigm emphasizing cognitive computing capability [1] , [2] , [3] , [4] , [5] , [6] . Synapse-motivated device networks make high power-efficiency and fast parallel processing feasible due to inherent architectural characteristics [7] , [8] , [9] , [10] , [11] , [12] . For instance, a simple signal—transmission action between neurons through a synapse only consumes a millionth of the energy required to execute the equivalent action in a traditional von Neumann computing system [13] . Non-volatile memory and history-dependent analogue-like states are two elemental characteristics for synapse-simulating devices [14] , [15] , [16] . Binary transition metal oxide-based two-terminal metal–insulator–metal memory resistance structures have been explored as the building blocks of neuromorphic systems [9] , [12] , [17] , [18] , [19] . Self-learning ability of the synapse is also a crucial attribute for cognitive computing [20] . Spike-timing-dependent plasticity (STDP), in which the change of synapse weight ( w ) is a function ( f 1 ) of the time difference between postneuron ( t post ) and preneuron ( t pre ) signals ( w=f 1 ( t post − t pre )), is one common self-learning process in human brains ( Fig. 1a ) [12] . Physically, the increase of synapse weight is manifested by augmentation of the quantity of neurotransmitters and dendritic receptors [21] . In biological systems, signal transmission and synapse learning are both generally regarded to occur concurrently in synapse-connected neuron pairs [22] . Current two-terminal metal–insulator–metal artificial synapses operate by separating the signal transmission and self-learning processes in time [8] , [9] . Three-terminal synaptic devices, being able to realize both functions simultaneously, therefore offer a promising solution for efficient synapse simulation [23] , [24] , [25] , [26] , [27] , [28] . 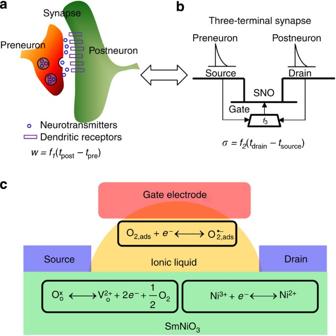Figure 1: Three-terminal nickelate synaptic transistor device. (a) In a neural synapse, the synapse weight (w), manifested by the quantity of neurotransmitters and dendritic receptors, is a function (f1) of the time difference between preneuron and postneuron spikes (tpost−tpre). (b) Three-terminal SmNiO3(SNO) transistor gated by ionic liquid with its channel conductance (σ) tuned by the time difference (tdrain−tsource) between source and drain spikes. Functionf3is applied to simulate the time difference between source and drain, which is manifested by the gate bias. (c) Proposed resistance modulation mechanism, in which oxidation and reduction of Ni species, through the creation/annihilation of oxygen vacancies in SNO channel by external electric field, is designed to enable SNO conductance switching. Figure 1: Three-terminal nickelate synaptic transistor device. ( a ) In a neural synapse, the synapse weight ( w ), manifested by the quantity of neurotransmitters and dendritic receptors, is a function ( f 1 ) of the time difference between preneuron and postneuron spikes ( t post − t pre ). ( b ) Three-terminal SmNiO 3 (SNO) transistor gated by ionic liquid with its channel conductance ( σ ) tuned by the time difference ( t drain − t source ) between source and drain spikes. Function f 3 is applied to simulate the time difference between source and drain, which is manifested by the gate bias. ( c ) Proposed resistance modulation mechanism, in which oxidation and reduction of Ni species, through the creation/annihilation of oxygen vacancies in SNO channel by external electric field, is designed to enable SNO conductance switching. Full size image Herein, we demonstrate a three-terminal rare-earth nickelate ( R NiO 3 , R =rare-earth element) thin-film transistor that mimics a biological synapse. By implementing such synaptic nickelate device, we successfully realize the first concurrent operation of signal transmission and STDP learning in correlated oxides, which provides a new opportunity and strategy to explore neuromorphic-correlated oxide electronics including programmable fluidic circuits. Device architecture and operation principle As correlated oxides with sharp thermally driven insulator–metal transition, nickelates are of interest in areas spanning from physics to electronics [29] , [30] . Figure 1b illustrates the schematic and operation of a synaptic transistor, in which the source and drain are analogues of the preneuron and postneuron terminals, respectively. Perovskite SmNiO 3 (SNO) is utilized as the channel material and is engineered to have properties of non-volatile memory, analogue states and learning function triggered by gate pulses. The metallic phase resistance of SNO is very sensitive to the stoichiometry [31] . Oxygen vacancies often lead to the destabilization of Ni 3+ , which is manifested by the increase of nickelates’ resistance in the metallic regime. Previously, the resistance modulation of bulk nickelates was achieved by adjusting the degree of oxygen deficiency during synthesis [31] , [32] , [33] . Recently, suppression or enhancement of the metallic phase of the nickelates was realized by introducing either tensile or compressive strain, which is believed to be able to regulate the Ni 3+ /Ni 2+ ratio [34] , [35] , [36] . The resistance modification from both methods is permanent and irreversible. Here, by modulating the stoichiometry of SNO by ionic liquid (IL) gating, the conductivity of the SNO is expected to be regulated in an in situ manner due to the stabilization and destabilization of Ni 3+ , which has been reported to have a fundamental role in the metal–insulator transition (MIT) mechanism of SNO [29] . This is fundamentally different from electrostatic modulation, in which the resistance tuning is limited by the extremely short screening length of correlated oxides and the resistance recovers relatively quickly upon the removal of gate bias [37] , [38] , [39] , [40] . In the synaptic device, the conductance ( σ ) of SNO emulates synapse weight and it is modified by gate pulses, which are received from a multiplexer and are a function ( f 3 ) (ref. 26 ) of the time difference between drain ( t drain ) (preneuron) and source ( t source ) (postneuron) pulses. In total, σ = f 2 ( t drain − t source ). Figure 1c illustrates the proposed conductance modulation mechanism. For synapse processes, the transmission and reception of ions are essential for non-volatile and analogue behaviours. We here simulate the synaptic process by the creation and annihilation of oxygen vacancies in the SNO channel by electrochemical reactions through the IL–SNO interface. Two principal chemical reactions occurring in this process are (1) and (2): The overall defect formation reaction within SNO can therefore be written as: The first reaction is commonly observed in oxides when an external bias is applied [41] , [42] , [43] , [44] , [45] . When oxygen leaves the SNO lattice, the Ni 3+ is destabilized and transforms to Ni 2+ , as shown in reaction (2), which leads to an increase of its resistance at the metallic state. In the ionic liquid, it is widely reported that oxygen gas can be reduced to superoxide by the oxygen reduction reaction as the IL itself undergoes electrochemical reactions [46] , [47] , [48] , [49] , Reaction (4) can happen when the oxygen gas reaches the gate electrode, which acts as a catalyst. Oxygen gas and this superoxide are usually stored in the IL in the form of O 2 and with the help of Pt catalyst. The superoxide can be oxidized back to oxygen gas when the amount of gas phase in the IL decreases [46] , [47] , [48] . The operation principle of the IL/SNO device can be summarized as: under positive gating, oxygen leaves SNO by forming oxygen vacancy leading to the reduction of Ni 3+ to Ni 2+ ; under negative gating, oxygen originally stored in IL in the gas form or oxidized back from the superoxide is incorporated into the SNO lattice to oxidize Ni 2+ back to Ni 3+ . The reversibility of reactions(1, 2, 3, 4), makes the reversible modulation of SNO’s conductance possible. It is expected that the nature of such electrochemical process could render the modulation of SNO’s conductance in a non-volatile and analogue manner. Preparation of SNO SNO, as the first nickelate with its insulator–metal transition temperature T IM (400 K) reaching above room temperature, is of great interest to explore integration of correlated oxides with conventional circuits [29] , [50] . Single-crystal Si with a thermal oxide (~60 nm thick) was used as the growth substrate. A combination of sputtering and ultrahigh pressure annealing was utilized for sample preparation (as the phase is not stable in ambient conditions) [51] . We synthesize samples in two ways: ceramic-target sputtering from a single Sm:Ni:3O target or metallic-target cosputtering from Sm and Ni targets, which allows us to have significant control over the grain size. Complete experimental details can be found in the Methods section. X-ray diffraction shows that the annealed phase is polycrystalline SNO ( Fig. 2a ), which can be viewed as a pseudocubic structure framed by tilted NiO 6 octahedra (inset of Fig. 2a ). Selective area electron diffraction captured from the SNO layer confirmed its phase (inset of Fig. 2b ). 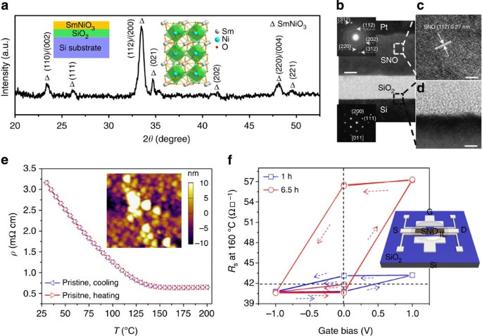Figure 2: Synthesis of SmNiO3films and transistor fabrication. (a) X-ray diffraction of a pristine SNO film on SiO2/Si. Insets show the layout of the film structure and the NiO6octahedra-framed orthorhombic SNO phase. (b) Cross-section transmission electron microscopy (TEM) image of SNO on SiO2/Si with inset images showing the electron diffraction patterns of both SNO and Si (scare bar, 20 nm);canddare high-resolution TEM images captured from SNO and Si layers, respectively (scare bar, 3 nm and 5 nm forcandd, respectively). (e) Resistivity–temperature measurements (cooling and heating) of the pristine SNO film showing no hysteresis in the phase transition. Roughness is determined to be ~5.0 nm, shown in inset atomic force microscopy image. (f) Sheet resistance–gate bias measurements with ±1 V bias for two durations (1.0 and 6.5 h) on the SNO film prepared by ceramic-target sputtering method. Inset shows the schematic of the ionic liquid-gated SNO device. Figure 2c shows the high-resolution transmission electron microscopy image of a local SNO region. The lattice spacing in this region (indexed by the dashed rectangle box) is ~0.27 nm, corresponding to the SNO (112) plane. Both selective area electron diffraction and high-resolution transmission electron microscopy acquired in the Si region ( Fig. 2d ) indicate that the top Si layer holds its single crystalline integrity and that it has an abrupt and smooth interface with the adjacent SiO 2 layer. Figure 2: Synthesis of SmNiO 3 films and transistor fabrication. ( a ) X-ray diffraction of a pristine SNO film on SiO 2 /Si. Insets show the layout of the film structure and the NiO 6 octahedra-framed orthorhombic SNO phase. ( b ) Cross-section transmission electron microscopy (TEM) image of SNO on SiO 2 /Si with inset images showing the electron diffraction patterns of both SNO and Si (scare bar, 20 nm); c and d are high-resolution TEM images captured from SNO and Si layers, respectively (scare bar, 3 nm and 5 nm for c and d , respectively). ( e ) Resistivity–temperature measurements (cooling and heating) of the pristine SNO film showing no hysteresis in the phase transition. Roughness is determined to be ~5.0 nm, shown in inset atomic force microscopy image. ( f ) Sheet resistance–gate bias measurements with ±1 V bias for two durations (1.0 and 6.5 h) on the SNO film prepared by ceramic-target sputtering method. Inset shows the schematic of the ionic liquid-gated SNO device. Full size image Figure 2e shows the resistivity–temperature ( R – T ) plot of the pristine SNO films. The resistivity in the metallic state is comparable to what is observed for epitaxial SNO grown on LaAlO 3 (ref. 38 ). The phase transition occurs at 140°C (identified by the slope change in the derivative plot, as shown in Supplementary Fig. S1 and discussed in Supplementary Note 1 ), which is slightly higher than the bulk value. The R – T curves during the cooling and heating stages overlap and no hysteresis was observed, which is also an indication of phase-pure characteristics of the SNO film, providing a robust platform for subsequent device investigation. A detailed discussion of the SNO MIT behaviour is further presented in Supplementary Fig. S1 and Supplementary Note 1 . In the inset of Fig. 2e is presented an atomic force microscopy image (1 × 1 μm) of the pristine SNO film prepared by the ceramic-target sputtering method. The surface roughness of the SNO film is ~5 nm and the grain size is several tens of nanometres. Resistance–gate bias hysteresis Photolithography was used to fabricate the three-terminal SNO device, as shown in the inset of Fig. 2f and Supplementary Fig. S2 and described in Supplementary Note 2 . The IL, which is composed of the anion tris(trifluoromethylsulfonyl)methide and the cation 1,2,3,4,5-pentamethylimidazolium (purchased from Covalent Associates Inc.), is utilized as the gate dielectric. Its high melting point (~120 °C) makes it chemically stable from room temperature to 200°C and therefore suitable for gating studies. Before electrical measurements, the IL is placed on top of the SNO channel and is baked at 160 °C in the liquid phase for 12 h under pure N 2 atmosphere to remove any water content. All subsequent measurements are performed in nitrogen flow unless otherwise indicated. Lateral gate bias is applied with reference to the grounded source terminal unless otherwise specified. By varying the gate voltage and its duration, a substantial resistance–gate bias hysteresis is observed reproducibly on the SNO device prepared by ceramic-target sputtering ( Fig. 2f ). At 160 °C, after applying a –1-V bias on the IL for 1 h, the sheet resistance of the SNO bar is reduced from 41.8 to 40.7 Ω per square. This resistance value remains stable for at least 1 h after bias is removed. We define this procedure as the starting point for the following gate bias cycling. Subsequently, a 1 h 1 V gate bias (blue line) increases the resistance from 40.6 to 43.2 Ω per square, and, alternately, a 6.5-h 1 V gate bias (red line) shifts it to 57.2 Ω per square. When the resistance reaches these two values, they essentially are stable with bias removed until long-duration negative pulses are applied. The original resistance can be recovered after several hours at −1 V bias, at which point the first cycle is defined to be finished. Then the same gating and measurement sequence as the first cycle is performed. It should be noted that all the measurements here are conducted at 160 °C, above T IM and the melting point of the IL. The second cycle closely repeats the first one for both gating durations (red and blue lines), indicating the reproducibility of this hysteresis phenomenon. Here, varying gating duration only changes the magnitude of the resistance–gate bias ( R – G ) loop but not its shape. The long timescales and hysteretic gating effect here suggests that such memristive and multistate behaviour in SNO is not from the electrostatic charge density modulation, such as that seen for epitaxial SNO devices fabricated on LaAlO 3 (ref. 38 ). Small grain size SNO transistor To reveal the IL gating effects in the full-temperature range above room temperature and the influence on the MIT characteristics of SNO prepared by the ceramic-target sputtering method, R – T measurements were performed on SNO devices gated at different voltages and durations. 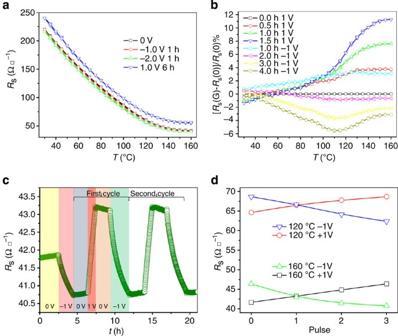Figure 3: Small grain size SmNiO3films. (a) Sheet resistance–temperature measurements under different gate bias voltages and durations. (b) Relative sheet resistance changes when device was gated by two bias polarities (1 and −1 V) in a sequence: 1 V for 0.0 h→1 V for 0.5 h→1 V for 1.0 h→1 V for 1.5 h→−1 V for 1.0 h→−1 V for 2.0 h→−1 V for 3.0 h→−1 V for 4.0 h. (c) Sheet resistance modulation versus time at two biases (1 and −1 V) and retention behaviours under zero bias. (d) Sheet resistance versus number of gate bias pulses at two polarities and two temperature points each. Each pulse duration is 30 min for 1 V and 1 h for −1 V. Figure 3a shows that under all circumstances, the SNO film still maintains its characteristic MIT feature. Negative bias of −1 V for 1 h and −2 V for 1 h both yield a downward shift of the R – T of SNO with the higher bias resulting in greater resistance modulation. When the bias polarity is switched to 1 V for 6 h, a substantial upward shift of the R – T is observed. To compare the relative change of sheet resistance at different temperatures, the SNO bar was gated at two polarities (1 and −1 V) for different durations. The sequence of the gating process is: 1 V for 0.0 h→1 V for 0.5 h→1 V for 1.0 h→1 V for 1.5 h→−1 V for 1.0 h→−1 V for 2.0 h→−1 V for 3.0 h→−1 V for 4.0 h ( Fig. 3b ). Positive polarity gating pulses produce a larger resistance change (up to 11% after 1.5 h gating), especially in the metallic phase region (160 °C); at negative bias it takes longer time to reach the same absolute value of resistance shift as positive bias. The relative resistance change gradually becomes smaller as we approach room temperature, indicating that modulation of the resistance of the insulating state of SNO is more difficult. Such observation of resistance modification of SNO shows similarity to the resistance modulation of bulk NdNiO 3 as a function of oxygen vacancies introduced during synthesis [33] . Figure 3: Small grain size SmNiO 3 films. ( a ) Sheet resistance–temperature measurements under different gate bias voltages and durations. ( b ) Relative sheet resistance changes when device was gated by two bias polarities (1 and −1 V) in a sequence: 1 V for 0.0 h→1 V for 0.5 h→1 V for 1.0 h→1 V for 1.5 h→−1 V for 1.0 h→−1 V for 2.0 h→−1 V for 3.0 h→−1 V for 4.0 h. ( c ) Sheet resistance modulation versus time at two biases (1 and −1 V) and retention behaviours under zero bias. ( d ) Sheet resistance versus number of gate bias pulses at two polarities and two temperature points each. Each pulse duration is 30 min for 1 V and 1 h for −1 V. Full size image Non-volatile memory behaviour is presented in Fig. 3c . Initially, the SNO film was kept for 2.5 h under zero bias, with its sheet resistance changing slowly due to small temperature drift. Then a negative bias of −1 V for 2 h was applied to reduce the resistance from 41.8 Ω per square in a nonlinear manner to 40.7 Ω per square. The resistance then holds this value for 2 h under zero gate bias. Further, the gate bias is switched to 1 V for 1 h and the resistance increases to 43.2 Ω per square linearly and drops slowly when the bias is removed over 2 h. Finally, it requires 2.7 h with −1 V bias to recover the resistance back to the low-resistance state, at which point the first cycle is finished. By following the same bias procedure, the second cycle measurement shows that this non-volatile memristive behaviour is nearly exactly reproducible. The multi-non-volatile states of SNO activated by the gate bias pulses are summarized in Fig. 3d . Each pulse of 1 V bias is held for 30 min at both 160 and 120 °C, whereas –1 V pulses are held for 1 h. Each pulse of positive gate polarity increases the resistance by ~1.5 Ω per square at 160 °C and slightly smaller at 120 °C. Conversely, each pulse of negative gate polarity yields a resistance drop of ~1.9 Ω per square at 160 °C with steep reduction in the first pulse and slower modulation in subsequent cycles. At 120 °C, a higher resistance drop rate is observed. The substantial non-volatile memory resistance property and analogue-like behaviour of the SNO film may allow for synaptic electronic applications. Large grain size SNO transistor It is generally known that the diffusion/migration rate of defects in oxides is very sensitive to the microstructure [52] . Atomic force microscopy and dark-field transmission electron microscopy images show that the grain size of SNO films prepared by the cosputtering method is a few hundred nanometres, whereas that of films from ceramic-target sputtering is a few tens of nanometres (see Supplementary Fig. S3 and Supplementary Note 3 ). To explore the effect of SNO microstructure on the non-volatile behaviour and analogue states, R – T measurements were performed on cosputtered SNO transistor devices. In Fig. 4a is presented R – T of an SNO gated by an IL along the following sequence: 1 V for 0.0 h→1 V for 0.25 h→1 V for 0.50 h→−1 V for 0.25 h→−1 V for 0.50 h→−1 V for 0.75 h→−2 V for 1.75 h. The characteristic R–T shape still holds at any gating bias for any pulsing duration. Similar to the ceramic-target-sputtered sample, in the metallic region, the upward shift triggered by the positive polarity is larger than the downward shift by a negative polarity, even when the negative bias magnitude is doubled. A substantial difference between cosputtered samples and ceramic-target-sputtered samples observed here is that the metallic sheet resistance modulation rate under 1 V gate bias is more than one order of magnitude higher in the former, possibly related to its distinct microstructure. This can be understood by the fact that grain boundaries can profoundly influence the diffusion characteristics in such ionic crystals [53] . The inset of Fig. 4a shows the resistance of the cosputtered SNO modulated by gate pulses at 160 and 120 °C (the duration for both 1 V and −1 V pulses is 15 min). The non-volatile and multistate behaviours of the SNO film are illustrated in Fig. 4b , in which 1 min pulses spaced 5 min apart of positive gate bias (in the sequence 0.5, 1.0, 1.5 and 2.0 V) and 30 s pulses spaced 5 min apart of negative gate bias (in the sequence −2.0, −1.5 and −1.0 V) are applied consecutively. At zero gate bias, the resistance stays constant or shifts significantly slower than with non-zero gate bias. 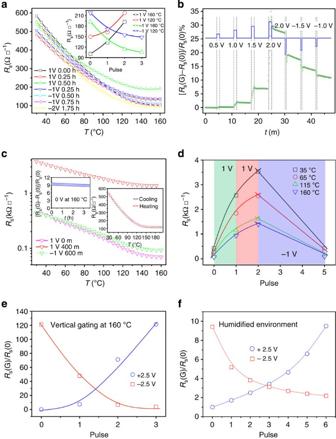Figure 4: Large grain size SmNiO3film. (a) Sheet resistance–temperature measurements under different gate biases and durations with the sequence: 1 V for 0.0 h→1 V for 0.25 h→1 V for 0.50 h→−1 V for 0.25 h→−1 V for 0.50 h→−1 V for 0.75 h→−2 V for 1.75 h. Inset shows the sheet resistance versus number of gate pulses at 120 and 160°C under 1 and −1 V. The pulse duration is 15 min for both 1 and −1 V biases. (b) Sheet resistance versus time for 1 min pulses spaced 5 min apart in the positive gate sequence 0.5, 1.0, 1.5 and 2.0 V and 30 s pulses spaced 5 min apart in the negative gate sequence −2.0, −1.5 and −1.0 V. (c) Sheet resistance–temperature at two biases (1 and −1 V) with very long pulse duration: 1 V for 400 min followed by −1 V for 10 h. Left inset shows the state retention characteristics after 200 min gating at 1 V. Right inset is the sheet resistance–temperature plots of the sample after several cycles of gating measurements. (d) Sheet resistance versus number of gate bias pulses at two polarities and four temperature points covering the metallic and insulating phases. Each pulse duration is 200 min for 1 V and 3 h for −1 V. (e) Sheet resistance modulation under vertical gate configuration for reduced gate-channel distance. Three orders faster modulation rate and resistance window is achieved compared with the lateral gating case. (f) Sheet resistance modulation under humidified N2, where one order faster resistance modulation speed is observed than in the dry N2case. Each pulse duration is 100 s for 2.5 V and 200 s for −2.5 V. Figure 4: Large grain size SmNiO 3 film. ( a ) Sheet resistance–temperature measurements under different gate biases and durations with the sequence: 1 V for 0.0 h→1 V for 0.25 h→1 V for 0.50 h→−1 V for 0.25 h→−1 V for 0.50 h→−1 V for 0.75 h→−2 V for 1.75 h. Inset shows the sheet resistance versus number of gate pulses at 120 and 160°C under 1 and −1 V. The pulse duration is 15 min for both 1 and −1 V biases. ( b ) Sheet resistance versus time for 1 min pulses spaced 5 min apart in the positive gate sequence 0.5, 1.0, 1.5 and 2.0 V and 30 s pulses spaced 5 min apart in the negative gate sequence −2.0, −1.5 and −1.0 V. ( c ) Sheet resistance–temperature at two biases (1 and −1 V) with very long pulse duration: 1 V for 400 min followed by −1 V for 10 h. Left inset shows the state retention characteristics after 200 min gating at 1 V. Right inset is the sheet resistance–temperature plots of the sample after several cycles of gating measurements. ( d ) Sheet resistance versus number of gate bias pulses at two polarities and four temperature points covering the metallic and insulating phases. Each pulse duration is 200 min for 1 V and 3 h for −1 V. ( e ) Sheet resistance modulation under vertical gate configuration for reduced gate-channel distance. Three orders faster modulation rate and resistance window is achieved compared with the lateral gating case. ( f ) Sheet resistance modulation under humidified N 2 , where one order faster resistance modulation speed is observed than in the dry N 2 case. Each pulse duration is 100 s for 2.5 V and 200 s for −2.5 V. Full size image To achieve larger sheet resistance modulation, longer gate pulses were applied to the SNO transistor. Figure 4c shows that after a 400-min pulse at 1 V, the whole R – T curve shifts upward with a relative resistance change of ~20 × in the metallic region (160°C) and a change of ~7 × in the insulating state (35 °C). The retention time of the high modulation state at 160 °C (after 1 V gating for 200 min) is demonstrated in the left inset of Fig. 4c , in which the resistance only dropped 5% after 3 h. Then by applying −1 V bias for 10 h, the R – T returns essentially to its original sate. Full R – T measurement from room temperature to 200 °C after several cycles of long-pulse gating indicates that the SNO film still maintains the MIT behaviour (right inset of Fig. 4c ). Resistance as a function of number of pulses presented in Fig. 4d demonstrates that orders of magnitude conductance modulation can be achieved in both insulating and metallic states when long pulses are applied. The asymmetry of the gating duration between positive and negative gate bias is related to the electrochemical nature of the conductance modulation. It is more favourable to have oxygen vacancies in SNO. Thus the conductance-modulation speed as a function of gate bias is asymmetric. The separation between gate electrode and SNO channel with IL as the gating medium is usually larger than in the case of typical solid-state gate dielectric thicknesses due to the difficulty of positioning the gate electrode. To investigate the effect of gate-channel distance on the resistance switching speed, under our current lateral gating configuration, we adjust the gate probe position and monitor the corresponding resistance switching rate, as shown in Supplementary Fig. S4 and described in Supplementary Note 4 . It shows that the resistance modulation rate increases more than one order when the gate-channel distance reduces accordingly. Adjusting gate-channel distance does not alter the magnitude of electric field across the IL–SNO interface due to the electric double layer. This finding thus indicates that ion diffusion in the IL is one of the rate-limiting processes during gating. To enable faster switching speed and a larger resistance window, we further reduce the gate-channel distance by vertically floating the gate electrode closely on the SNO channel. As shown in Fig. 4e , such vertical gating configuration with the shortest gate-channel distance (likely of the order of few tens of micrometres) that we can obtain gives us a three orders higher switching speed and resistance window than the lateral gating configuration. The duration of each pulse is 10 s for positive gating and 20 s for negative gating. The resistance switching speed/window under different gating pulses of fixed biases is presented in Supplementary Fig. S5 and described in Supplementary Note 5 . One, therefore, expects that even faster gating speed may be realized once the current IL gating medium (with the ion diffusion length in micrometre scale) is substituted by a solid-state dielectric layer (with the ion diffusion length in nanometre scale). To investigate the effect of atmosphere on the device performance and help understand the gating mechanism, the resistance modulation experiments were also conducted under humidified N 2 in the lateral gating configuration ( Fig. 4f ). We intentionally introduce moisture in the testing atmosphere by flowing the N 2 though a 60 °C de-ionized (DI) water bubbler before N 2 reaches the sealed probe station. It is found that the resistance modulation rate is approximately one order higher than that under dry N 2 in lateral gating geometry. This is consistent with the observation that water or protons can serve as catalysts to facilitate the oxygen reduction reaction process in IL [54] , [55] . Role of defects in SNO resistance modulation The SNO films were characterized by X-ray photoelectron spectroscopy to understand the mechanisms leading to the resistance modulation. X-ray photoelectron spectroscopy was conducted to reveal the role of oxygen defects in the IL gating process (see Supplementary Fig. S6a and Supplementary Note 6 ). For both the ceramic-target-sputtered and cosputtered samples, the Ni 2p 3/2 peak shifts to lower binding energy after 1 V gating. This indicates the increase of Ni 2+ concentration and reduction of Ni 3+ , which could be due to the loss of oxygen in SNO [31] , [56] , [57] . To simulate the oxygen vacancy evolution process, a pristine SNO film was annealed in air at 300 °C under atmospheric pressure. Our thermodynamic calculations show that such conditions are favourable for the transition of Ni 3+ to Ni 2+ , which must accompany the loss of oxygen [51] . Various annealing experiments (see Supplementary Fig. S6b and Supplementary Note 6 ) illustrate that indeed the sheet resistance continuously rises as the annealing time increases, which agrees with our hypothesis on the effect of oxygen vacancy defects in modulating the channel resistance. Based on all the above observations, we summarize the detailed process of resistance switching in the IL-gated SNO film, as presented in the Supplementary Note 7 . Synaptic properties simulated by SNO transistor To emulate neural stimulation and mimic the potentiation and depression processes, consecutive short gate pulses (periodic 10 ms gate pulses spaced 1 s apart) of 2.5 and −2.5 V were applied with short gate-channel distance in the vertical gating configuration ( Fig. 5a ). Approximately 1,500 cycles of negative pulses raised the sheet conductance of SNO by 1,000% and it required ~900 positive pulses to reduce the sheet conductance back to the initial value. The results suggest that the SNO device can potentially simulate synaptic analogue action with reasonable switching speed in the present configuration. To further increase the potentiation and depression rates, larger magnitude gate pulses may be applied. Solid-state electrolyte materials such as fast-ion conductors in thin films form with nanometre-scale thickness (ion diffusion length), which can sustain high potentials, can also be explored in future and would be of interest in this temperature range [58] . To realize STDP functionality, the source and drain of the SNO device can be connected to a multiplexer that converts the time difference between postneuron spikes (drain) and preneuron spikes (source) to a voltage pulse. The magnitude of the voltage pulse is proportional to the time difference while its duration is maintained at 10 s. Detailed circuitry realizing this functionality can be found in the Supplementary Fig. S7 , Supplementary Table S1 and Supplementary Note 8 . Here, we simulate the output of such a multiplexer by applying gate pulses of varying magnitude, corresponding to time differences between preneuron and postneuron spikes, using a standard voltage supply. 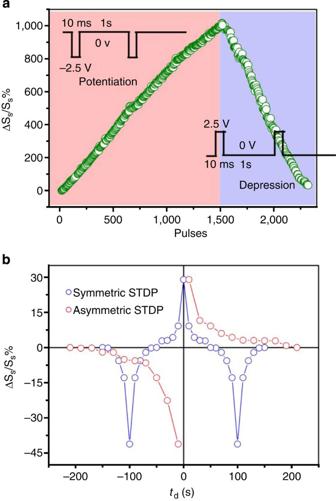Figure 5: Simulation of synaptic properties. (a) Sheet conductance modulation of SmNiO3under repeated potentiation (2.5 V for 10 ms spaced 1 s apart) and depression (−2.5 V for 10 ms spaced 1 s apart) gate pulses with vertical gate configuration. (b) Demonstration of asymmetric and symmetric synaptic spike-timing-dependent plasticity synapse functions in a nickelate device (tdstands for time difference). Figure 5b shows the measured percentage change of sheet conductance of an SNO device under such simulated time differences. For asymmetric STDP function, when the drain spike is before the source spike, the conductance (synaptic weight) decreases. When the drain spike is after the source spike, a reverse modulation is observed. In both cases, when the time difference is small, the conductance change is greater. Such modulation scenario mimics neural synaptic STDP behaviour in various biological systems. By programming the shape of the source spike (see Supplementary Fig. S7 , Supplementary Table S1 and Supplementary Note 8 ), symmetric synaptic STDP function is also achieved ( Fig. 5b ). The successful demonstration of STDP in a three-terminal nickelate device introduces a novel material system and innovative working principle for developing neuromorphic devices. Figure 5: Simulation of synaptic properties. ( a ) Sheet conductance modulation of SmNiO 3 under repeated potentiation (2.5 V for 10 ms spaced 1 s apart) and depression (−2.5 V for 10 ms spaced 1 s apart) gate pulses with vertical gate configuration. ( b ) Demonstration of asymmetric and symmetric synaptic spike-timing-dependent plasticity synapse functions in a nickelate device ( t d stands for time difference). Full size image We herein reveal that controlling oxygen vacancy in correlated nickelate through a liquid/solid interface could enable conductance modulation and realize non-volatile and analogue states, which are required in synaptic devices. Defect creation and its consequence on electrical properties is closely linked to the crystal structure of the oxides and cation valence stability. The increase of oxygen vacancy in SNO (under positive gating) leads to an increase in resistivity in the metallic regime, which is similar to experimental observations in VO 2 (refs 45 , 59 ). This is understandable as introducing defects in metallic phase provides more electronic scattering sites. In the insulating regime, introducing oxygen vacancies modulates resistivity non-monotonously, which is related to the increase in divalent character of Ni–O bonds. In the case of VO 2 , introducing more oxygen vacancies leads to the reduction of its resistivity, which is related to the evolution of reduced cation species. Our study presents the first demonstration of synaptic action in three-terminal correlated oxide devices that can operate above room temperature and be integrated onto silicon platforms. By taking advantage of the deterministic role of stoichiometry on the electrical properties of correlated nickelates, conductance can be modulated in a non-volatile and analogous way. To enable faster operation of the synapse and larger modulation of the synaptic weight, high potentiation or depression potential spikes and solid-state electrolytes such as fast-ion conductors could be explored in the future. With liquids, this can allow realization of programmable fluidic circuits and open up new frontiers in correlated electron systems. Synthesis of SNO Growth of polycrystalline SNO was realized in a sputtering process with ultrahigh pressure annealing. Before sputtering, the substrate SiO 2 /Si was cleaned by acetone, isopropanol and DI water and then dried by N 2 gas. We utilized two sputtering methods for the deposition of SNO films: (1) with a single Sm:Ni:3O-sintered ceramic target; (2) cosputtering with Sm and Ni metal targets. For both the ceramic-target sputtering and cosputtering, the growth was conducted at 5 mTorr in a constant flow of 40/10 sccm Ar/O 2 mixture with the substrate at room temperature. The radio frequency power for the Sm:Ni:3O target was 200 W. The DC power for the Ni target was adjusted to 75 W and radio frequency power for the Sm target was 150 W to obtain a ~1:1 Sm:Ni cation ratio, as determined by energy-dispersive X-ray spectroscopy. Growth time ranged from 30 min to a few hours to vary the film thickness. The as-sputtered samples were then transferred to a home-built high-pressure vessel system. Detailed instrumentation information and thermodynamic conditions for phase formation could be found in the study by Jaramillo et al . [51] The vessel was then inserted into a tube furnace and ramped to 500 °C for 24 h at 1,500 psi pure O 2 . After annealing, the sample was cleaned by acetone, isopropanol and DI water and then dried by N 2 . Device fabrication and electrical measurement With standard photolithography, three-terminal SNO transistor devices were fabricated. Dilute hydrogen chloride (3:1 H 2 O: HCl) was used to etch SNO. Pt electrodes of 100 nm thickness were prepared by DC sputtering for Ohmic electrical contact and good mechanical adhesion. Electrical measurement was conducted with a Keithley 2635A source meter in a probe station (Materials Development Corporation) with 200 sccm pure N 2 continuously flowing at ambient pressure. Gate bias was applied with a Keithley 230 voltage supply. Before electrical measurement, the ionic liquid-covered device was baked at 160 °C for 12 h in N 2 atmosphere to remove water contamination. How to cite this article: Shi, J. et al . A correlated nickelate synaptic transistor. Nat. Commun. 4:2676 doi: 10.1038/ncomms3676 (2013).